Activation of allylic esters in an intramolecular vinylogous kinetic resolution reaction with synergistic magnesium catalysts Kinetic resolution (KR) of racemic starting materials is a powerful and practical alternative to prepare valuable enantiomerically enriched compounds. A magnesium-catalyzed kinetic resolution based on a designed intramolecular vinylogous Michael reaction is disclosed. Here we show a synergistic catalytic strategy based on the development of chiral ligands. Substrates containing linear allylic ester structures are designed and synthesized to construct key [6.6.5]-tricyclic chiral skeletons via this kinetic resolution process. Detailed mechanistic studies reveal a rational mechanism for the current intramolecular vinylogous KR reaction. The desired direct intramolecular asymmetric vinylogous Michael reaction of linear allylic esters is realized in high efficiency and enantioselectivity with the synergistic catalytic system. Catalytic nonenzymatic kinetic resolution (KR) of racemic starting materials that mediates the selective reaction of one enantiomer has been recognized as a powerful and practical alternative to preparing valuable enantiomerically enriched compounds, and found wide applications in both academia and industry [1] , [2] , [3] , [4] . Most documented nonenzymatic KR reactions use intermolecular pathways, with the selection of one appropriate reactive partner to finish the desired KR process. In contrast, the development of intramolecular KR reactions have been relatively less investigated, as they require an ideal match between the designed substrates and small molecule catalysts [5] , [6] , [7] , [8] , [9] , [10] , [11] , [12] , [13] , [14] . Herein, we design an intramolecular vinylogous Michael reaction of linear allylic esters for a KR process to build chiral parallel [6.6.5]-tricyclic skeletons, which exist in many natural products and pharmaceutically active compounds, such as Juglocombin B, Glaziovianol, and some COX-2 and ubiquitin-connected enzymes inhibitors (Fig. 1 ) [15] , [16] , [17] , [18] , [19] . This reaction also represents one alternative to asymmetric dearomatizative pathways of 1-naphthols [20] , [21] , [22] , [23] , [24] , [25] , [26] . Fig. 1: Reaction design and related compounds containing the key [6.6.5]-tricyclic skeletons. a Synergistic catalytic strategy for the direct intramolecular asymmetric vinylogous Michael reaction. b Related natural products and pharmaceutically active compounds containing the tricyclic skeletons. Full size image Compared with other linear allylic carbonyl compounds, simple linear allylic esters are less reactive and less investigated in asymmetric reactions [27] , [28] , [29] . To date, there are still very few studies on the direct activation of linear allylic esters in catalytic asymmetric reactions. Moreover, the α-position of linear allylic esters might dominate the C-C bond formation process especially in the reaction with Michael acceptors [30] , [31] , [32] . In most cases, activated or modified allylic esters are often necessary to overcome the low reactivity of these types of substrates [33] , [34] , [35] , [36] , [37] , [38] , [39] . For example, in the widely used vinylogous Mukaiyama reaction, it is necessary to prepare the unstable dienolsilanes in a separate step [33] , [34] , [35] , [36] , [37] . Only until very recently, the Yin group reported direct asymmetric vinylogous aldol reactions of allylic esters using chiral copper catalysts and additive bases [40] . They also achieved the asymmetric alkynylogous aldol reaction by an optimized propargyl copper(I) catalytic method [41] . These reactions are highly efficient and ideal for the direct use of allylic esters as feedstock. However, the direct catalytic asymmetric intramolecular vinylogous reaction of allylic esters has not yet been achieved [42] , [43] , [44] . Herein, by developing a synergistic in situ generated magnesium catalytic strategy [45] , [46] , [47] , [48] , [49] , [50] , [51] , [52] , [53] , [54] , [55] , we successfully employ the vinylogous Michael reaction of linear allylic esters in a rationally designed intramolecular KR process (Fig. 1 ). Reaction optimization Initially, we designed and synthesized the allylic ester 1a for the intramolecular KR reaction. Bifunctional diols containing amine groups (Fig. 2 ) were selected as chiral ligands for sequencing process to the magnesium catalysts. 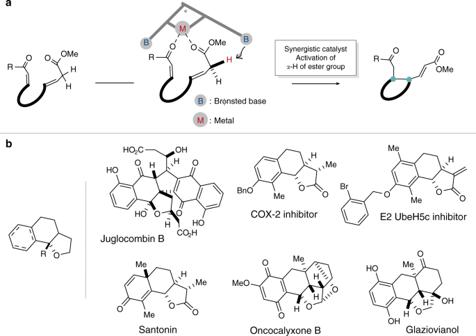Fig. 1: Reaction design and related compounds containing the key [6.6.5]-tricyclic skeletons. aSynergistic catalytic strategy for the direct intramolecular asymmetric vinylogous Michael reaction.bRelated natural products and pharmaceutically active compounds containing the tricyclic skeletons. The desired intramolecular vinylogous Michael reaction proceeded primarily from one enantiomer, and resulted in enantiomerically enriched parallel [6.6.5]-tricyclic skeletons (Table 1 ). Different tertiary amines-modified diol ligands were screened, and pyrrolidine-modified ligand L1 had better resolution results compared with those of other tertiary amine groups (Table 1 , entries 1-5). Further modification at the 6,6’-position of the BINOL skeletons led to the successful synthesis of a series of bifunctional chiral ligands (Fig. 2 , L7 - L10 ). These modifications dramatically affected the efficiency of the magnesium catalysts, and the introduction of chloride was identified as giving the best results for the intramolecular vinylogous KR reaction (Table 1 , entry 10). The synthetic route for ligand L10 is illustrated in Fig. 2 . Fig. 2: Selection and development of bifunctional chiral ligands and related synthetic methods. a Bifunctional chiral ligands screened in the optimization process. b Synthetic method of chiral ligand L10 and related X-ray analysis. Full size image Table 1 Optimization of the vinylogous KR reaction a . Full size table Substrate scope Next, we investigated the scope for the intramolecular vinylogous KR reaction (Fig. 3 ). The magnesium catalytic system proved to be robust for the selective conversion of different alkyl-substituted substrates, furnished the desired KR process smoothly under mild conditions. A variety of substituted [6.6.5]-tricyclic rings were obtained in high enantioselectivities (92:8-98.5:1.5 er), and the enantiomerically enriched allylic esters 1* were recovered in satisfactory results. Substrates with aryl groups also finished the designed KR process, although relatively higher catalyst loading (20 mol%) was required (Fig. 3 ). The absolute configuration of the resolution adducts was determined by the X-ray crystallographic analysis of 2b (Fig. 3 ). Fig. 3: Substrate scope of the KR reaction. See Supplementary Information for the detail experiment processes. All yields shown were based on isolated products. er values were determined by chiral HPLC analysis. s = ln[(1 − C)(1 − ee)]/ln[(1 − C)(1 + ee)], where ee = ee 1a* /100, ee 1a* = (R 1a* – S 1a* )/(R 1a* + S 1a* )*100, C is monitored by HPLC analysis and calculated according to C = ee 1a* /(ee 1a* + ee 2a ). Full size image Subsequently, different benzohexene ketone motifs were introduced into the allylic ester substrates and used in the vinylogous KR reaction. Polycyclic structures were established under the magnesium catalytic system. Electron-withdrawing or electron-donating groups were under trial in the KR process (Fig. 4 ). Fig. 4: Further extensions of the substrate scope of the KR reaction. All yields shown were based on isolated products. er values were determined by chiral HPLC analysis. Full size image Interestingly, it was observed that for substrate 1t , bearing two Michael receptor sites, the vinylogous Michael reaction occurred during the KR process to form the quaternary stereocenter, and generate the bridged-ring adduct 2t [56] . In addition, some of 1t* was recovered at a moderate er value. The common cyclization adduct 2t’ was not observed under the catalytic system, instead, some undetermined decomposition products were generated, resulting in the relatively lower yields of 2t and 1t* (Fig. 5 ). Fig. 5: Site-selective results of the substrate 1t in the KR reaction. Isolated yields are reported. Full size image Transformations The vinylogous KR reaction was then carried out at the gram scale and transformations of the recovered 1a * were conducted. As illustrated in Fig. 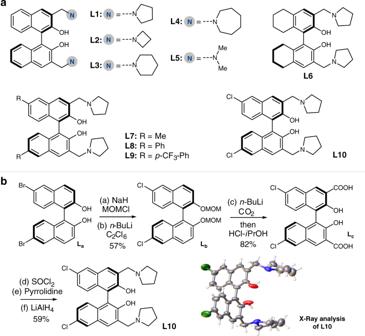Fig. 2: Selection and development of bifunctional chiral ligands and related synthetic methods. aBifunctional chiral ligands screened in the optimization process.bSynthetic method of chiral ligandL10and related X-ray analysis. 6 , the recovered substrate 1a* formed the cyclization adduct 2a’ , by treatment with NaOMe. Under photocatalytic conditions lead to the polycyclic product 3 after finishing the [2 + 2] cyclization process (Fig. 6 ) [57] , [58] , [59] , [60] . Fig. 6: Gram scale trial and related transformation of 1a*. 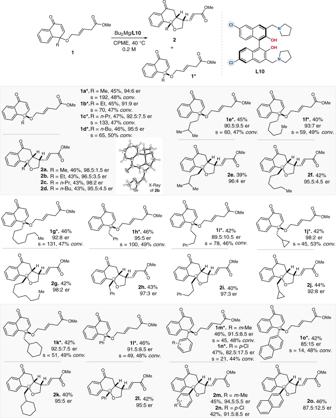Fig. 3: Substrate scope of the KR reaction. See Supplementary Information for the detail experiment processes. All yields shown were based on isolated products. er values were determined by chiral HPLC analysis. s = ln[(1 − C)(1 − ee)]/ln[(1 − C)(1 + ee)], where ee = ee1a*/100, ee1a*= (R1a*– S1a*)/(R1a*+ S1a*)*100, C is monitored by HPLC analysis and calculated according to C = ee1a*/(ee1a*+ ee2a). a Gram scale experiments of the KR process. b Transformations of the isolated chiral allylic ester 1a* . Full size image To our pleasure, the rearomatization reaction was easily realized by treating 2a with p -toluenesulfonic acid under mild conditions, This reaction can be used for the formal construction of γ-arylation adduct 4 with high enantioselectivity and good yield (Fig. 7 ). Fig. 7: Transformations of resolution products. Conditions: a with CuI (2.5 mol%), Pd(PPh 3 ) 4 (2.5 mol%), Et 3 N (2.0 equiv) in DMF at room temperature. b with PPh 3 (20 mol%), Pd(OAc) 2 (10 mol%), Et 3 N (2.0 equiv) in THF/CH 3 CN at room temperature. c with PPh 3 (6 mol%), PdCl 2 (PPh 3 ) 2 (3 mol%), K 2 CO 3 (1.5 equiv) in Dioxane at 80 °C. d with Pd(PPh 3 ) 4 (5 mol%), K 2 CO 3 (2.0 equiv) in H 2 O/ Dioxane reflux for 24 h. Full size image Additional transformations of the tricyclic rings were performed for this central [6.6.5] skeleton to form compounds that might be useful for pharmaceutical investigations [15] , [16] , [17] , [18] , [19] . We introduced different functional groups or heterocyclic structures to the central skeletons by selected cross-coupling reactions. These transformations were carried out by established transition-metal mediated coupling reactions as illustrated in Fig. 7 . Mechanistic studies To investigate mechanistic aspects of the intramolecular vinylogous KR reaction, we performed a variety of mechanistic experiments. We first performed control experiments to identify the reason for the high efficiency of the bifunctional magnesium catalyst. 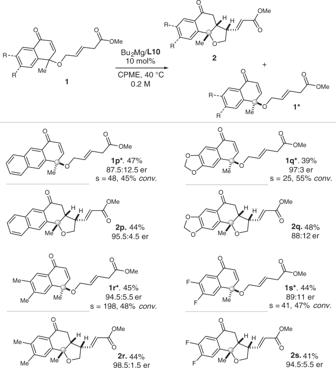Fig. 4: Further extensions of the substrate scope of the KR reaction. All yields shown were based on isolated products. er values were determined by chiral HPLC analysis. As illustrated in Fig. 8 , simple in situ generated magnesium catalyst from BINOL cannot promote the intramolecular vinylogous reaction (Fig. 8 , a). Introduction of tertiary amine at high loading mediated generation of the trace cyclization adduct, and the combined use of the BINOL-Mg catalyst and tertiary amine activated the allylic ester 1a to form intramolecular vinylogous Michael adduct 2a . These results indicate the magnesium center and the Brønsted base can synergistically activate the designed allylic ester substrate. The developed bifunctional magnesium catalyst is more effective in the vinylogous KR reaction even with the ligand L12 with lower Brønsted basicity (Fig. 8 , a). Subsequently, studies of nonlinear effects revealed the synergistic catalyst interacts with the bidentate substrate as a mono-species (Fig. 8 , b) [61] , [62] . 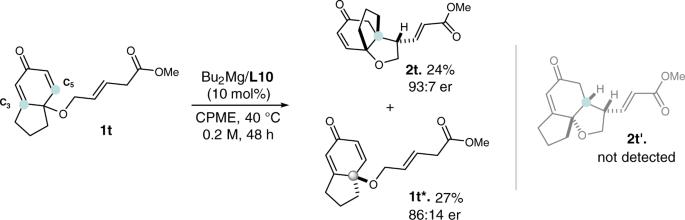Fig. 5: Site-selective results of the substrate 1t in the KR reaction. Isolated yields are reported. Further investigations on ESI experiments of the initial reaction complexes clearly indicated the coordination results of the immediately introduced bidentate substrate 1a to the bifunctional magnesium catalyst, which is well in accordance with the calculated results (Fig. 8 , c). Fig. 8: Mechanistic studies for the synergistic catalyst in the KR reaction. a Control experiments of the KR reaction under different catalytic conditions. b Nonlinear effects studies of the KR reaction. c ESI experiments of the initial reaction complexes to investigate the activation mode. Full size image Proposed mechanism Combination with the mechanistic insights, a possible mechanism cycle of the intramolecular vinylogous KR reaction is proposed (Fig. 9 ). The bifunctional magnesium catalyst is smoothly generated from L10 and Bu 2 Mg after the neutralization process, then the bidentate substrate coordinates to the magnesium center and the tertiary amine synergistically promotes enolation of the allylic ester. At the same time, the bidentate coordination results in synchronous activation of the Michael receptor to promote the intramolecular vinylogous reaction in the well-controlled chiral environment (Fig. 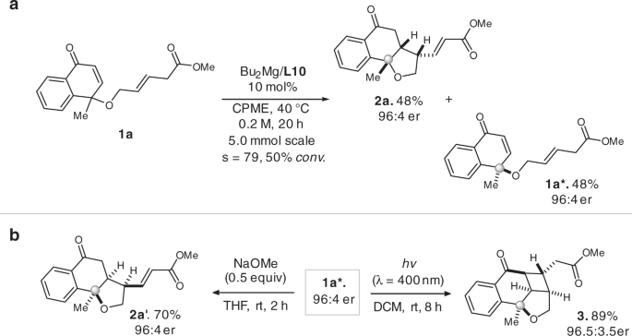Fig. 6: Gram scale trial and related transformation of 1a*. aGram scale experiments of the KR process.bTransformations of the isolated chiral allylic ester1a*. 9 , II and III). Finally, the protonation process and the entry of another molecule of 1a lead to the release of the KR product 2a . Fig. 9: Proposed mechanism. Possible reaction mechanism for the synergistic magnesium catalyst promoted KR reaction. 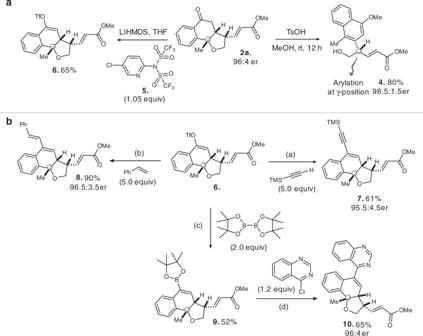Fig. 7: Transformations of resolution products. Conditions:awith CuI (2.5 mol%), Pd(PPh3)4(2.5 mol%), Et3N (2.0 equiv) in DMF at room temperature.bwith PPh3(20 mol%), Pd(OAc)2(10 mol%), Et3N (2.0 equiv) in THF/CH3CN at room temperature.cwith PPh3(6 mol%), PdCl2(PPh3)2(3 mol%), K2CO3(1.5 equiv) in Dioxane at 80 °C.dwith Pd(PPh3)4(5 mol%), K2CO3(2.0 equiv) in H2O/ Dioxane reflux for 24 h. Full size image In summary, we have accomplished a direct catalytic asymmetric intramolecular vinylogous Michael reaction. Bifunctional chiral ligands were developed to generate synergistic magnesium catalysts. Using the designed allylic ester substrates, the KR process successfully led to the expected [6.6.5]-tricyclic key skeletons. Several transformations were conducted to give types of chiral polycyclic structures and derivatives of the [6.6.5]-tricyclic skeletons, as well as the enantioselective γ-arylation adduct. Combinational mechanistic insights, including control experiments, nonlinear effects studies and relative ESI investigations, led to the proposal of a possible mechanism of this intramolecular vinylogous KR reaction. Further developments of the reported synergistic magnesium catalyst in asymmetric reactions are underway in our laboratory. General procedure for the vinylogous KR reaction To a stirred solution of L10 (10.42 mg, 0.02 mmol) in CPME (0.5 mL) was added Bu 2 Mg (20 μL, 1.0 M in heptane, 0.02 mmol) under an argon atmosphere, the mixture was then stirred at room temperature for 30 min to generate the catalyst. The substrate 1 (0.2 mmol) in CPME (0.5 mL) was quickly added to the flask containing the in situ generated magnesium catalyst. After the addition, the reaction was stirred at 40 °C and analyzed by TLC. The reaction was quenched with saturated NH 4 Cl and extracted with CH 2 Cl 2 . 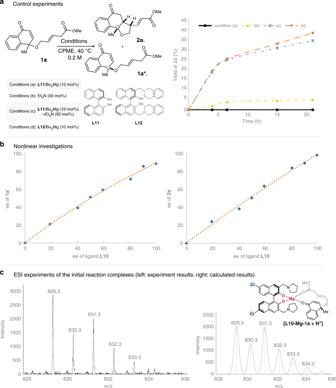Fig. 8: Mechanistic studies for the synergistic catalyst in the KR reaction. aControl experiments of the KR reaction under different catalytic conditions.bNonlinear effects studies of the KR reaction.cESI experiments of the initial reaction complexes to investigate the activation mode. 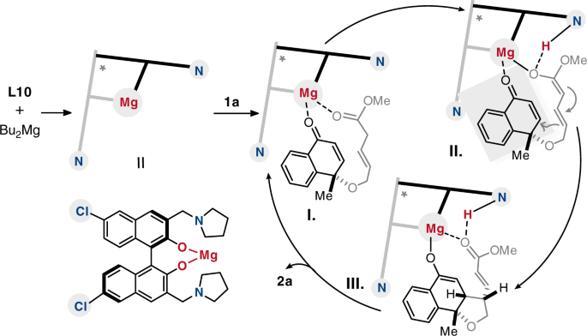Fig. 9: Proposed mechanism. Possible reaction mechanism for the synergistic magnesium catalyst promoted KR reaction. The organic layer was dried over anhydrous Na 2 SO 4 and concentrated under vacuum. Then the residue was purified by column chromatography to afford the product 1 * and 2 .